Epigenetic changes induced by in utero dietary challenge result in phenotypic variability in successive generations of mice 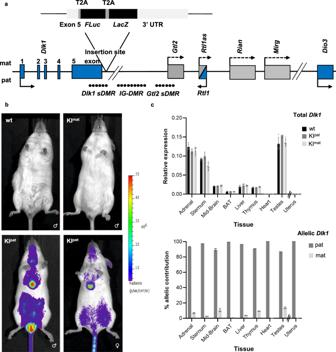Fig. 1: Generation and characterisation of reporter mice for imprintedDlk1expression. aSchematic of the mouseDlk1-Dio3imprinted locus showing reporter insertion. Three differentially methylated regions (DMRs) that regulate imprinted expression of the cluster are indicated (closed circles represent methylated CpGs,IG-DMR,Dlk1 sDMRandGtl2 sDMR) and the position of maternally expressed (light grey) and paternally expressed (blue) genes are shown. Arrows depict transcriptional direction, with solid lines representing protein-coding genes and striped lines representing non-coding transcripts. In theDlk1-FLucLacZreporter line,firefly Luciferase(FLuc) andβ–galactosidase(LacZ) were knocked into the endogenousDlk1locus, with T2A sites, downstream of exon 5.bBioluminescence (BL, blue) was detected in 8-week-old (P56) male (lower panel, left) and female mice (lower panel, right) after paternal transmission of the reporter (KIpat). Strong BL signal was evident in the thymus, central sternum and testes. Minimal signal was detected in animals after maternal reporter transmission (KImat, upper panel, right) or in wild-type animals (wt, upper panel, left).cDlk1expression analysed by QRT-PCR (upper panel) was compared in different tissues from P56 male mice that inherited the reporter paternally (KIpat, dark grey), maternally (KImat, light grey), or in non-transgenic controls (wt, black). Uterus samples from age-matched female mice were also analysed. Expression levels were normalized toβ-Actin,18SandHprtexpression (bars show the geometric mean of relative expression, error bars represent the geometric standard deviation (geometric SD)). Genotype had no significant effect onDlk1expression (Two-way ANOVA on delta-Ct values (Tissuep< 0.0001, Genotypep= 0.86, Interactionp= 0.98);N= 4 + 4 + 4 individual mice). AllelicDlk1analysis in KImatmice (lower panel), using primers that distinguish the reporter from the wt allele, showed a strong bias for paternal allele expression (dark grey) compared to maternal allele expression (light grey). (Bars indicate the mean contribution from each allele ±SD;N= 4 + 4 individual mice). Source data are provided as a Source Data file. Transmission of epigenetic information between generations occurs in nematodes, flies and plants, mediated by specialised small RNA pathways, modified histones and DNA methylation. Similar processes in mammals can also affect phenotype through intergenerational or trans-generational mechanisms. Here we generate a luciferase knock-in reporter mouse for the imprinted Dlk1 locus to visualise and track epigenetic fidelity across generations. Exposure to high-fat diet in pregnancy provokes sustained re-expression of the normally silent maternal Dlk1 in offspring (loss of imprinting) and increased DNA methylation at the somatic differentially methylated region ( sDMR ). In the next generation heterogeneous Dlk1 mis-expression is seen exclusively among animals born to F1-exposed females. Oocytes from these females show altered gene and microRNA expression without changes in DNA methylation, and correct imprinting is restored in subsequent generations. Our results illustrate how diet impacts the foetal epigenome, disturbing canonical and non-canonical imprinting mechanisms to modulate the properties of successive generations of offspring. Epigenetic gene regulation, and the processes that enable information that is not strictly encoded by DNA to be transmitted to offspring, is the subject of intense study in model organisms [1] , [2] , [3] , [4] , [5] , [6] , [7] , [8] and in man [9] , [10] . Genomic imprinting is an epigenetically regulated process that restricts mammalian gene expression in a parent-of-origin-specific manner [11] , [12] . Mono-allelic gene expression is initiated by differential DNA methylation of parental germlines but is often reinforced postfertilisation by the acquisition of additional epigenetic features that help sustain appropriate allelic expression (or silencing) within somatic tissues [13] , [14] , [15] . As a group, imprinted genes are critical for controlling embryonic growth and placental development [13] , [14] , [16] and have key roles later in postnatal life, where they influence metabolism, neurogenesis and behaviour [17] , [18] , [19] . The expression of imprinted genes is tightly regulated and subtle changes in expression often lead to profound changes in phenotype [17] , [20] , [21] . Dlk1 is a prototypic paternally expressed, imprinted gene that is broadly expressed in the mid-gestation embryo but becomes increasingly restricted in the adult to subpopulations of cells in the adrenal and pituitary glands, skeletal muscle, liver and brain [22] , [23] , [24] , [25] , [26] . Paternally restricted expression of Dlk1 is associated with reciprocal expression of maternal Gtl2 ( Meg3 ), Rian ( Meg8 ), anti-sense Rtl1 ( Rtl1as ), as well as clusters of intergenic microRNAs ( Mirg ) that collectively comprise one of the largest microRNA (miR) clusters in the genome [27] . Molecular studies have shown that imprinting of the Dlk1-Dio3 region is primarily regulated by a differentially methylated region (DMR), the IG-DMR , that shows selective methylation on the paternally inherited allele. Localised methylation across the Dlk1 somatic DMR ( sDMR ) and Gtl2 sDMR occurs after fertilization and reinforces allelic marking to ensure expression of Dlk1 and Gtl2 from paternal and maternal alleles respectively [24] , [28] , [29] . Luciferase-based imaging offers a powerful non-invasive approach to visualise gene expression longitudinally in mammals [30] , [31] . We have previously shown that targeting luciferase into endogenous imprinted genes, such as Cdkn1c , enables allelic expression to be monitored in living mice throughout their lifespan. These reporter mice have also been used to show that in utero exposure to chromatin-modifying drugs, or dietary stress, can induce a sustained loss of imprinting (LOI) in offspring [30] . Here we ask whether diet-induced deregulation of imprinting can be inherited across generations. Using a bespoke mouse luciferase reporter for allelic Dlk1 expression, we show that F1 animals that were exposed to a maternal high-fat diet (HFD) in utero experience a sustained loss of Dlk1 imprinting. F2 offspring born to exposed F1 mothers exhibit deregulated and ectopic expression of Dlk1 . We show that this intergenerational change in phenotype stems from alterations in the transcriptional profile of oocytes from embryos that were exposed to HFD in utero. Dlk1-FlucLacZ reporter mice show imprinted Dlk1 expression We generated a mouse reporter in which firefly luciferase ( FLuc ) and β-galactosidase ( LacZ ) were knocked into the 3’UTR of the endogenous Dlk1 gene. The targeting strategy (Fig. 1a and methods) employed T2A sites to generate Dlk1-FLucLacZ RNA species under the control of the Dlk1 promoter, that upon translation and self-cleavage at T2A sites, produce individual luciferase, β-galactosidase and Dlk1 proteins. To confirm that luciferase activity accurately reports Dlk1 expression in these mice, we performed a series of bioluminescence (BL) imaging, immunohistology and molecular analyses. The engineered Dlk1 reporter allele showed faithful paternal expression [17] , [26] with BL signal exclusively detected in Dlk1-FLucLacZ adult mice that inherited the reporter paternally (KI pat , Fig. 1b ) and evident in the brain, abdomen, testes, liver, adrenal glands and central sternum. No BL signal was seen in Dlk1-FLucLacZ mice inheriting the reporter maternally (KI mat ), or in wild-type (wt) control animals. Tissue-specific and allelic Dlk1 expression in the Dlk1-FLucLacZ reporter mice was verified by QRT-PCR. As shown in Fig. 1c (upper panel), Dlk1 transcript levels were similar in reporter and non-transgenic animals, consistent with minimal locus disruption. As anticipated, transgene-derived Dlk1 expression was detected in adrenal, midbrain, liver, testes, and in brown adipose tissue (BAT), but not in heart or uterine tissue. A strong bias in expression from the paternal allele was confirmed in each of these tissues (Fig. 1c , lower panel) consistent with the imprinted expression of Dlk1 that has been reported previously [22] , [32] , [33] , [34] . To further validate these molecular analyses, we examined Dlk1 immunolabelling and LacZ staining on adult tissue from control (wt) and reporter ( Dlk1-FLucLacZ ) mice. As anticipated, Dlk1 is readily detected in pituitary and adrenal tissues, but not in kidney or heart (Fig. S1a ). Similarly, in KI pat reporter mice Dlk1 labelling was evident in the pituitary, adrenal, and liver tissue (Fig. S1b , left column) and undetected in heart. Examination of sequential sections of KI pat tissues stained for LacZ showed a close correspondence between LacZ stain and Dlk1 distribution. No LacZ staining was evident in equivalent tissues derived from adult KI mat or wt mice (Fig. S1b , right-hand columns). These data highlight the fidelity of the Dlk1-FLucLacZ mouse line to report tissue-specific and imprinted Dlk1 expression. Fig. 1: Generation and characterisation of reporter mice for imprinted Dlk1 expression. a Schematic of the mouse Dlk1-Dio3 imprinted locus showing reporter insertion. Three differentially methylated regions (DMRs) that regulate imprinted expression of the cluster are indicated (closed circles represent methylated CpGs, IG-DMR , Dlk1 sDMR and Gtl2 sDMR ) and the position of maternally expressed (light grey) and paternally expressed (blue) genes are shown. Arrows depict transcriptional direction, with solid lines representing protein-coding genes and striped lines representing non-coding transcripts. In the Dlk1-FLucLacZ reporter line, firefly Luciferase ( FLuc ) and β–galactosidase ( LacZ ) were knocked into the endogenous Dlk1 locus, with T2A sites, downstream of exon 5. b Bioluminescence (BL, blue) was detected in 8-week-old (P56) male (lower panel, left) and female mice (lower panel, right) after paternal transmission of the reporter (KI pat ). Strong BL signal was evident in the thymus, central sternum and testes. Minimal signal was detected in animals after maternal reporter transmission (KI mat , upper panel, right) or in wild-type animals (wt, upper panel, left). c Dlk1 expression analysed by QRT-PCR (upper panel) was compared in different tissues from P56 male mice that inherited the reporter paternally (KI pat , dark grey), maternally (KI mat , light grey), or in non-transgenic controls (wt, black). Uterus samples from age-matched female mice were also analysed. Expression levels were normalized to β-Actin , 18S and Hprt expression (bars show the geometric mean of relative expression, error bars represent the geometric standard deviation (geometric SD)). Genotype had no significant effect on Dlk1 expression (Two-way ANOVA on delta-Ct values (Tissue p < 0.0001, Genotype p = 0.86, Interaction p = 0.98); N = 4 + 4 + 4 individual mice). Allelic Dlk1 analysis in KI mat mice (lower panel), using primers that distinguish the reporter from the wt allele, showed a strong bias for paternal allele expression (dark grey) compared to maternal allele expression (light grey). (Bars indicate the mean contribution from each allele ±SD; N = 4 + 4 individual mice). Source data are provided as a Source Data file. Full size image To verify that DNA methylation was correctly maintained in these reporter mice we performed bisulphite analysis across the Dlk1 sDMR , IG-DMR and Gtl2 sDMR , comparing Dlk1-FLucLacZ KI pat and wt samples of adult liver. Methylation levels were indistinguishable at each of the Dlk1 DMR regions analysed (Fig. S1c ). An independent method was also used to verify these results. As shown in Fig. S1d pyrosequencing analysis at the Dlk1 sDMR confirmed similar levels of DNA methylation in Dlk1-FLucLacZ KI pat , Dlk1-FLucLacZ KI mat and wt samples. Taken together these results support the view that Dlk1-FLucLacZ accurately reports endogenous Dlk1 expression and that reporter insertion at the Dlk1-Dio3 locus had not substantially altered the methylation of regulatory DMRs. BL imaging studies performed during pregnancy revealed abdominal reporter signal in pregnant mice carrying embryos with a paternally inherited Dlk1 -reporter (Fig. 2a , left) and dissection and ex vivo imaging confirmed expression in E11.5 embryos (Figs. 2b, c and S2a ). Transiently, from E11.5 to E14.5 a weaker signal was seen in embryos with a maternally inherited Dlk1 -reporter, but this was extinguished by E17.5 (Fig. 2c ). Temporal reinforcement of mono-allelic Dlk1 expression during development is consistent with prior reports [32] , [35] , [36] . To examine tissue-specific reporter expression in developing embryos, whole-mount staining for LacZ and optical projection tomography was performed on E11.5 embryos (Fig. S2b , Movies S1 – 3 ). LacZ staining showed abundant Dlk1-FLucLacZ reporter expression in KI pat embryos with signal prominent in the forebrain, cartilage, developing lung, liver, pancreas and tongue (Fig. S2b ), consistent with the developmental expression of Dlk1 that has been previously reported [22] , [37] . Within the KI pat forebrain, immunolabelling confirmed that luciferase expression (red) was restricted to a subset of cells co-labelled with anti-Dlk1 antibody (green, Fig. S2c ). Fig. 2: Inheritance of imprinted Dlk1 reporter expression in embryos and across generations. a BL signal (blue) detected in Dlk1-FLucLacZ pregnancies arising from KI pat (left) and KI mat (right) transmission showed greater surface signal in KI pat pregnancies (E11.5). b Quantification of BL signal (Flux) detected in E11.5 Dlk1-FLucLacZ embryos following dissection, demonstrating higher levels of signal from KI pat than KI mat embryos. BL signal in wt and KI mat embryos is shown as a percentage of the average KI pat signal (number of embryos ( N ) indicated in table; One-way ANOVA on log-transformed data ( p < 0.0001); results of Holm-Šídák’s multiple comparisons follow-up test are shown for comparisons to wt mice, and between KI pat /KI mat mice as indicated: ****adjusted p ( p adj) < 0.0001). Source data are provided as a Source Data file. c BL imaging of embryos at different stages (E11.5, E14.5 and E17.5) showed progressive reduction in signal (blue) in both KI pat (left panel) and KI mat (right panel) through gestation; signal was readily detected in E11.5 and E14.5 KI pat and KI mat embryos, but at later stages (E17.5) was only seen after paternal transmission. Signal intensity scales are equalised between images. d Transmission of mono-allelic imprinted Dlk1 reporter expression in four generations (F0, F1, F2, F3); upon paternal inheritance of Dlk1-FLucLacZ the reporter was expressed (blue), while maternal inheritance resulted in reporter silencing (white). Imprinting was predictably re-set across generations, through both germlines (a minimum of two independent litters were analysed per generation and reciprocal cross). Full size image To verify that imprint erasure and re-setting occurs correctly in the Dlk1-FLucLacZ reporter line, we tracked BL activity in animals established from reciprocal crosses spanning four generations ( N > 6 per reciprocal cross and generation). 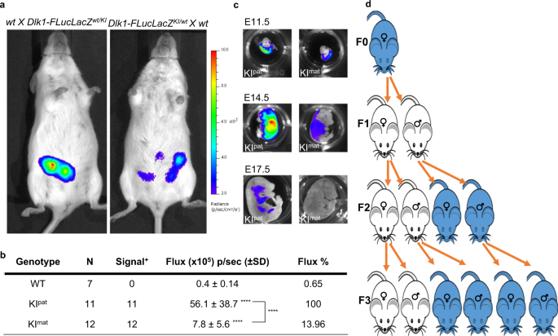Fig. 2: Inheritance of imprintedDlk1reporter expression in embryos and across generations. aBL signal (blue) detected inDlk1-FLucLacZpregnancies arising from KIpat(left) and KImat(right) transmission showed greater surface signal in KIpatpregnancies (E11.5).bQuantification of BL signal (Flux) detected in E11.5Dlk1-FLucLacZembryos following dissection, demonstrating higher levels of signal from KIpatthan KImatembryos. BL signal in wt and KImatembryos is shown as a percentage of the average KIpatsignal (number of embryos (N) indicated in table; One-way ANOVA on log-transformed data (p< 0.0001); results of Holm-Šídák’s multiple comparisons follow-up test are shown for comparisons to wt mice, and between KIpat/KImatmice as indicated: ****adjustedp(padj) < 0.0001). Source data are provided as a Source Data file.cBL imaging of embryos at different stages (E11.5, E14.5 and E17.5) showed progressive reduction in signal (blue) in both KIpat(left panel) and KImat(right panel) through gestation; signal was readily detected in E11.5 and E14.5 KIpatand KImatembryos, but at later stages (E17.5) was only seen after paternal transmission. Signal intensity scales are equalised between images.dTransmission of mono-allelic imprintedDlk1reporter expression in four generations (F0, F1, F2, F3); upon paternal inheritance ofDlk1-FLucLacZthe reporter was expressed (blue), while maternal inheritance resulted in reporter silencing (white). Imprinting was predictably re-set across generations, through both germlines (a minimum of two independent litters were analysed per generation and reciprocal cross). 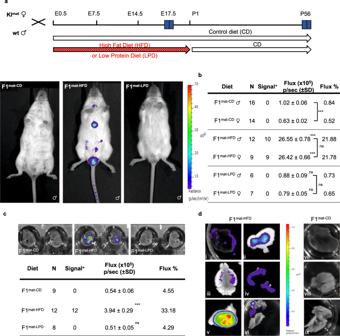Fig. 3: Exposure to high fat diet in utero results in loss ofDlk1imprinting in offspring. aTemporal scheme of experimental breeding, dietary regime and bioluminescent image analysis. Offspring inheritingDlk1-FLucLacZmaternally (KImat) were generated by mating wt males with heterozygousDlk1-FLucLacZfemales; upon detection of a vaginal plug pregnant females were maintained on a control (CD) diet or switched to low protein diet (LPD), or high fat diet (HFD), for the duration of the pregnancy. At birth, all animals were maintained on CD and BL imaging was performed on reporter offspring at the times indicated (E17.5 and postnatal day 56). Increased BL signal (blue) was evident in P56 mice that had been exposed to gestational HFD (F1mat-HFD, middle image), as compared to either CD or LPD-exposed animals (F1mat-CD, F1mat-LPD, left and right, respectively).bAbdominal bioluminescence signal was significantly increased in F1mat-HFDoffspring (P56) as compared to F1mat-CDor F1mat-LPD. BL signal in F1mat-HFDanimals was less than that in dietary control animals that inherited the reporter paternally (KIpat-CD), suggesting a partial release of silencing. (Number of animals (N) indicated in table; Two-way ANOVA on log-transformed data (Dietp< 0.0001; Sexp= 0.049; Interactionp= 0.0046); results of Holm-Šídák’s multiple comparisons follow-up test are shown: ***padj = 0.0004, ****padj < 0.0001, ns=not significant). Source data are provided as a Source Data file.cBL signal (blue) in E17.5 embryos from F1mat-HFD, F1mat-LPDand F1mat-CDare compared (upper panel) and quantified (lower panel showing Flux levels relative to KIpat-CDcontrols). BL signals were significantly higher in F1mat-HFDthan F1mat-LPDand F1mat-CDembryos. (Number of embryos (N) indicated in table; One-way ANOVA on log-transformed data (p< 0.0001); results of Dunnett’s multiple comparisons follow-up test comparing to F1mat-CDembryos are shown: ****padj < 0.0001, ns=not significant). Source data are provided as a Source Data file.dBL signal (blue) detected ex vivo in organs of male P56 F1mat-HFDanimals (left panels: i- liver, ii- white adipose, iii- brain, iv- uterus (taken from female animals), v- testes, vi- brown adipose tissue). Control tissues from P56 F1mat-CDanimals (right panels: vii- liver, viii- brain, ix- brown adipose) are shown for comparison. Figure 2d illustrates these results, showing that epigenetic inheritance in the Dlk1-FLucLacZ colony followed the expected pattern for a paternally expressed imprinted gene. Collectively these results reaffirm that Dlk1-FLucLacZ mice are reliable models of imprinted Dlk1 expression. HFD in pregnancy causes loss of Dlk1 imprinting in offspring Foetal exposure to maternal diet low in protein or high in fat, can induce long-lasting changes in gene expression, physiology and behaviour in offspring [10] , [38] , [39] , [40] . We showed previously that exposure to low protein diet in utero provokes sustained LOI of the maternally expressed imprinted gene Cdkn1c in offspring [30] . To examine whether the paternally expressed Dlk1 gene was sensitive to dietary challenge, we crossed Dlk1-FLucLacZ females with wt males and exposed pregnant dams to either control diet (CD), low protein diet (LPD) or high-fat diet (HFD) throughout pregnancy, as outlined in Fig. 3a . Gestational exposure to altered diet resulted in modest changes in dam and embryonic weights (Figs. S3a and S3b ), consistent with the dietary model [41] , [42] , [43] , [44] , [45] , [46] . Maternally transmitted Dlk1-FLucLacZ is predicted to be silent in offspring derived from these crosses and consistent with this all F1 animals that had been exposed to CD (F1 mat-CD ) in utero showed BL signal at near background levels (Figs. 3a, b ). Imprinted expression was also maintained in all F1 animals that had been exposed to LPD (F1 mat-LPD ) in utero. In sharp contrast, exposure to HFD resulted in F1 animals (F1 mat-HFD ) that expressed maternally-derived Dlk1 (19/21, Figs. 3a, b ). This LOI was observed in mature male and female F1 mat-HFD offspring, long after gestational exposure and after being switched back to a normal control diet. LOI was also evident in HFD-exposed embryos at E17.5 (Fig. 3c ), at a time in gestation where Dlk1 expression was shown to be exclusively derived from the paternal allele (Fig. 2c ). In adults, maternally derived Dlk1 -reporter signal was evident in dissected brain, liver, thyroid, testes and adipose tissues of F1 mat-HFD animals (Fig. 3d , images i-vi), as compared to F1 mat-CD (Fig. 3d , images vii-ix). BL signal was generally detected in tissues where paternally-derived Dlk1 expression would be predicted, although ectopic expression was seen in the uterus. Fig. 3: Exposure to high fat diet in utero results in loss of Dlk1 imprinting in offspring. a Temporal scheme of experimental breeding, dietary regime and bioluminescent image analysis. Offspring inheriting Dlk1-FLucLacZ maternally (KI mat ) were generated by mating wt males with heterozygous Dlk1-FLucLacZ females; upon detection of a vaginal plug pregnant females were maintained on a control (CD) diet or switched to low protein diet (LPD), or high fat diet (HFD), for the duration of the pregnancy. At birth, all animals were maintained on CD and BL imaging was performed on reporter offspring at the times indicated (E17.5 and postnatal day 56). Increased BL signal (blue) was evident in P56 mice that had been exposed to gestational HFD (F1 mat-HFD , middle image), as compared to either CD or LPD-exposed animals (F1 mat-CD , F1 mat-LPD , left and right, respectively). b Abdominal bioluminescence signal was significantly increased in F1 mat-HFD offspring (P56) as compared to F1 mat-CD or F1 mat-LPD . BL signal in F1 mat-HFD animals was less than that in dietary control animals that inherited the reporter paternally (KI pat-CD ), suggesting a partial release of silencing. (Number of animals ( N ) indicated in table; Two-way ANOVA on log-transformed data (Diet p < 0.0001; Sex p = 0.049; Interaction p = 0.0046); results of Holm-Šídák’s multiple comparisons follow-up test are shown: *** p adj = 0.0004, **** p adj < 0.0001, ns=not significant). Source data are provided as a Source Data file. c BL signal (blue) in E17.5 embryos from F1 mat-HFD , F1 mat-LPD and F1 mat-CD are compared (upper panel) and quantified (lower panel showing Flux levels relative to KI pat-CD controls). BL signals were significantly higher in F1 mat-HFD than F1 mat-LPD and F1 mat-CD embryos. (Number of embryos ( N ) indicated in table; One-way ANOVA on log-transformed data ( p < 0.0001); results of Dunnett’s multiple comparisons follow-up test comparing to F1 mat-CD embryos are shown: **** p adj < 0.0001, ns=not significant). Source data are provided as a Source Data file. d BL signal (blue) detected ex vivo in organs of male P56 F1 mat-HFD animals (left panels: i- liver, ii- white adipose, iii- brain, iv- uterus (taken from female animals), v- testes, vi- brown adipose tissue). Control tissues from P56 F1 mat-CD animals (right panels: vii- liver, viii- brain, ix- brown adipose) are shown for comparison. Full size image Dlk1 LOI in F1 mat-HFD animals was associated with a selective increase in DNA methylation at the Dlk1 sDMR (with an increased trend at the Gtl2 sDMR , but not the IG-DMR ) in affected tissues such as liver and BAT (exemplified in Fig. 4a ), and with increased gene expression across the entire Dlk1 cluster (Figs. 4b and S3b ). Detailed molecular analyses confirmed significant increases in total Dlk1 expression in liver, mid-brain and testes of adult F1 mat-HFD animals as compared to matched F1 mat-CD controls (Fig. 4c , upper panel), while Dlk1 expression remained extremely low in tissues such as adult heart. Allelic analysis confirmed maternally-derived Dlk1 expression in adrenal glands, midbrain, BAT, liver, testes and uterus of adult F1 mat-HFD animals (Fig. 4c , lower panel), consistent with prior bioluminescent data. Fig. 4: Altered DNA methylation and allelic mis-expression of Dlk1 in offspring exposed to HFD in utero. a DNA bisulphite methylation analysis at Dlk1 sDMR , IG-DMR and Gtl2 sDMR in liver (upper) and brown adipose tissue (BAT) (lower) from representative male P56 F1 mat-CD and F1 mat-HFD animals. In liver and BAT, hypermethylation was detected at Dlk1 sDMR , increased methylation was observed at the Gtl2 sDMR (not statistically significant), but IG-DMR was unchanged. Closed circles indicate methylated CpGs, open circles un-methylated CpGs. Each row represents an individual clone. Percentages indicate total methylation level of the region from two wt and two KI mat animals. (Kolmogorov-Smirnov test comparing clonal methylation levels, using Holm-Šídák’s correction for multiple comparisons: ** p adj < 0.0055, **** p adj = 6 × 10 −6 , ns=not significant). Source data are provided as a Source Data file. 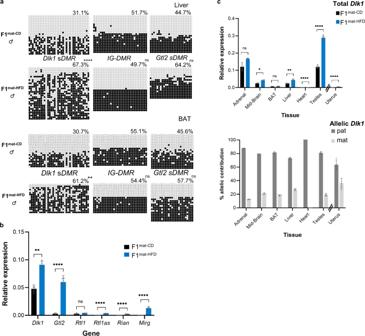Fig. 4: Altered DNA methylation and allelic mis-expression ofDlk1in offspring exposed to HFD in utero. aDNA bisulphite methylation analysis atDlk1 sDMR,IG-DMRandGtl2 sDMRin liver (upper) and brown adipose tissue (BAT) (lower) from representative male P56 F1mat-CDand F1mat-HFDanimals. In liver and BAT, hypermethylation was detected atDlk1 sDMR, increased methylation was observed at theGtl2 sDMR(not statistically significant), butIG-DMRwas unchanged. Closed circles indicate methylated CpGs, open circles un-methylated CpGs. Each row represents an individual clone. Percentages indicate total methylation level of the region from two wt and two KImatanimals. (Kolmogorov-Smirnov test comparing clonal methylation levels, using Holm-Šídák’s correction for multiple comparisons: **padj < 0.0055, ****padj = 6 × 10−6, ns=not significant). Source data are provided as a Source Data file.bGene expression (QRT-PCR) at theDlk1-Dio3cluster in the liver of male P56 F1mat-HFD(blue) and F1mat-CD(dark grey) animals. Expression levels for this single tissue comparison were normalised toβ-Actinexpression. (Bars show the geometric mean of relative expression with geometric SD;N= 4 + 4 individual mice; unpaired two-sidedt-tests on delta-Ct values with Holm-Šídák’s correction for multiple comparisons: **padj = 0.0067, ****padj < 0.0001, ns=not significant). Source data are provided as a Source Data file.cDlk1expression (QRT-PCR, upper panel) in different tissues from P56 male mice exposed to either control (F1mat-CD, black) or high-fat diet (F1mat-HFD, blue). Uterus samples from age-matched female mice were also analysed. Expression levels were normalised toβ-Actin,18SandHprt. (Bars show the geometric mean of relative expression with geometric SD;N= 4 + 4 individual mice; Two-way ANOVA on delta-Ct values (Tissuep< 0.0001, Dietp< 0.0001, Interactionp< 0.0001); results of Holm-Šídák’s multiple comparisons follow-up test for effect of diet in each tissue are shown: *padj = 0.013, **padj = 0.0042, ****padj < 0.0001, ns=not significant). AllelicDlk1analysis in F1mat-HFDmice (lower panel), using primers that distinguish the reporter from the wt allele, showed a reduced contribution for paternal allele expression (dark grey) when compared to maternal allele expression (light grey). (Bars indicate the mean contribution from each allele ±SD;N= 4 + 4 individual mice). Source data are provided as a Source Data file. b Gene expression (QRT-PCR) at the Dlk1-Dio3 cluster in the liver of male P56 F1 mat-HFD (blue) and F1 mat-CD (dark grey) animals. Expression levels for this single tissue comparison were normalised to β-Actin expression. (Bars show the geometric mean of relative expression with geometric SD; N = 4 + 4 individual mice; unpaired two-sided t -tests on delta-Ct values with Holm-Šídák’s correction for multiple comparisons: ** p adj = 0.0067, **** p adj < 0.0001, ns=not significant). Source data are provided as a Source Data file. c Dlk1 expression (QRT-PCR, upper panel) in different tissues from P56 male mice exposed to either control (F1 mat-CD , black) or high-fat diet (F1 mat-HFD , blue). Uterus samples from age-matched female mice were also analysed. Expression levels were normalised to β-Actin , 18S and Hprt . (Bars show the geometric mean of relative expression with geometric SD; N = 4 + 4 individual mice; Two-way ANOVA on delta-Ct values (Tissue p < 0.0001, Diet p < 0.0001, Interaction p < 0.0001); results of Holm-Šídák’s multiple comparisons follow-up test for effect of diet in each tissue are shown: * p adj = 0.013, ** p adj = 0.0042, **** p adj < 0.0001, ns=not significant). Allelic Dlk1 analysis in F1 mat-HFD mice (lower panel), using primers that distinguish the reporter from the wt allele, showed a reduced contribution for paternal allele expression (dark grey) when compared to maternal allele expression (light grey). (Bars indicate the mean contribution from each allele ±SD; N = 4 + 4 individual mice). Source data are provided as a Source Data file. Full size image Dlk1 misregulation in F2 offspring To investigate whether HFD-induced alteration of Dlk1 was transmitted to subsequent generations, we examined F2 mice derived from crosses between F1 mat-HFD females and wt males (F2 mat-HFD , Fig. 5a ). In this setting maternal inheritance is predicted to ensure Dlk1 silencing, however, BL signal was detected in most F2 mat-HFD offspring, as illustrated for a litter of eleven animals (Fig. 5b ) in which seven were transgenic (KI mat ). BL signal distribution suggested that Dlk1 misexpression was variable among F2 mat-HFD animals, consistent with a partial LOI (Fig. 5c ). Molecular analyses of liver, heart and mid-brain samples from individual F2 mat-HFD mice confirmed heterogeneity in male and female offspring that were derived from F1 mat-HFD females and suggested ectopic expression of Dlk1 in the heart (Figs. 5d and S4a ). This was confirmed by immunolabelling of individual heart tissue, with Dlk1 detected in three out of four F2 mat-HFD mice, as compared to negative F2 mat-CD control tissue (Fig. S4b ). Importantly, a strong correlation between elevated levels of Dlk1 detected by molecular and immunohistochemical approaches was noted in individual F2 mat-HFD animals (Figs. S4a and S4b ). To exclude that Dlk1 expression showed intrinsic variation between generations, we compared expression in F1 and F2 offspring exposed to CD. As shown in Fig. S4c , Dlk1 expression in different tissues remained unchanged between generations under CD conditions, and minimal expression was detected in the heart. Together these data support the view that gestational exposure to HFD results in heterogenous and ectopic expression of Dlk1 in F2 offspring. Fig. 5: Exposure-induced changes to Dlk1 imprinting are transmitted to F2 offspring. a Schematic for generational studies following HFD exposure. Gestationally exposed animals ( Dlk1-FLucLacZ F1 mat-HFD ) were bred with wt (CD-fed) mates, maintained on CD, and F2 and F3 offspring examined. b BL signal (blue) in F2 offspring (F2 mat-HFD ) derived from F1 HFD-exposed females. Signal was variable and ectopic. c Abdominal BL signal in P56 F2 mat-HFD males (open-circles) and females (filled-circles), from six F1 mat-HFD females and wt CD males (litters 1–5, no litter from female 6) or two F1 mat-HFD males and wt CD females (litters 7–8). KI mat-CD and KI pat-CD signal shown for comparison. Litter 4 is represented in ( b ). Source data are provided as a Source Data file. d Dlk1 expression (QRT-PCR, left) in tissues from P56 males (uterus from females) whose mothers were exposed in utero to CD (F2 mat-CD , black) or HFD (F2 mat-HFD , red). Expression normalised to β-Actin , 18S and Hprt (bars show geometric mean with geometric SD; N = 4 + 4 individual mice; Two-way ANOVA on delta-Ct values (Tissue p < 0.0001, Diet p = 0.002, Interaction p < 0.0001); Holm-Šídák’s multiple comparisons follow-up test for diet in each tissue: **** p adj < 0.0001, ns=not significant). Allelic Dlk1 analysis in F2 mat-HFD mice (right) showed reduced paternal (dark grey) versus maternal (light grey) expression bias, compared to control conditions (bars indicate mean allelic contribution ±SD; N = 4 + 4 individual mice). Source data are provided as a Source Data file. e Bisulphite analysis in male P56 F2 mat-HFD liver showed Dlk1 sDMR hyper-methylation, increased IG-DMR methylation ( p adj = 0.078) and slightly reduced Gtl2 sDMR methylation, compared to F1 mat-CD (Fig. 4a ). Closed circles: methylated CpG, open circles: un-methylated CpG. Rows show individual clones from a representative individual, percentages indicate total methylation from two animals. (Kolmogorov-Smirnov test comparing clonal methylation levels, using Holm-Šídák’s correction for multiple comparisons: * p adj = 0.025, *** p adj = 0.0001, ns=not significant). Source data are provided as a Source Data file. f Summary of altered Dlk1 expression following gestational HFD. Dlk1 is silent (white) when transmitted maternally and expressed (blue) when transmitted paternally. Gestational HFD exposure provokes LOI in F1 offspring (blue, box). F1 females transmit altered Dlk1 expression to F2 offspring (blue, box), whereas F1 males and F2 females transmit Dlk1 appropriately. Full size image Detailed molecular analysis revealed that despite the partial loss of Dlk1 imprinting seen in F2 mat-HFD animals (Fig. 5d , right), overall levels of Dlk1 expression were generally lower in tissues such as adrenal glands, midbrain, liver and testes, than in controls (Fig. 5d , left). Altered DNA methylation across the Dlk1-Dio3 locus was also detected in F2 mat-HFD somatic tissue, as illustrated in Fig. 5e . In F2 offspring generated from reciprocal crosses (F1 mat-HFD males x wt females), Dlk1 reporter expression was consistent with normal paternal inheritance and imprinting (Fig. 5c , litters 7 and 8). One explanation for the LOI in second-generation offspring from HFD-exposed females is that in utero exposure affects the developing epigenome of oocytes contained within developing female embryos, as well as affecting F1 somatic tissue. This scenario evokes an intergenerational mode of epigenetic inheritance, rather than requiring trans-generational mechanisms [5] and predicts that normal imprinting would be restored in subsequent generations (Fig. 5f ). Consistent with this possibility, BL signal was undetectable in all F3 transgenic animals derived from LOI-affected F2 mat-HFD dams (as exemplified in Fig. S5a ), although levels of Dlk1 -associated gene expression were generally lower in HFD-exposed offspring (F3 mat-HFD and F2 mat-HFD ) as compared with CD-exposed (F2 mat-CD ) controls (Fig. S5b ). Gestational HFD alters transcription in developing oocytes To better understand the basis of ectopic Dlk1 reporter expression in F2 mat-HFD offspring, we asked whether DNA methylation was perturbed in the gametes of F1 mat-HFD mice. As predicted, F1 mat-HFD sperm showed DNA methylation exclusively at the IG-DMR , with hypo-methylation at Dlk1 sDMR and Gtl2 sDMR (Fig. S6 ). F1 mat-HFD oocytes were collected individually and processed for parallel genome-wide single-cell bisulphite sequencing and single-cell RNA-seq (scM&Tseq) (quality control shown in Figs. S7a and S7b ) [47] , [48] . In both groups the anticipated bimodal pattern of DNA hypo- and hypermethylated domains in oocytes [48] , [49] was retained, with a broadly similar profile assessed over 100-CpG windows ( r = 0.984) (Figs. S8a and S8b ). While differences in methylation were detected in 439 differentially methylated 100-CpG tiles (representing approximately 0.2% of genomic tiles) these were dispersed across the genome (Fig. S8c ) and principal component analysis (PCA) indicated no obvious separation of oocytes from different groups (Fig. S8a ). Among the imprinted gametic DMRs, high levels of methylation of maternal gDMRs and low levels of methylation of paternal gDMRs were well preserved in F1 mat-HFD oocytes (Fig. 6a ) and we did not detect significantly increased variation or anomalous gDMR methylation of F1 mat-HFD oocytes as compared with F1 mat-CD (Figs. S8d and S8e ). At the Dlk1-Dio3 imprinted domain itself, the IG-DMR domain remained similarly hypo-methylated in F1 mat-CD and F1 mat-HFD groups, while the Dlk1 sDMR and Gtl2 sDMR showed minimal changes in methylation in F1 mat-HFD oocytes (Fig. 6b ) that were not statistically significant. The lack of changes in DNA methylation levels at the Dlk1-Dio3 imprinted domain make it unlikely that this is responsible for the highly penetrant maternal transmission of ectopic Dlk1 expression seen after in utero HFD exposure. Fig. 6: Germline DMRs in single MII oocytes from F1 females are unaffected by dietary exposure but show an altered transcriptional programme. a Heatmap representing mean DNA methylation levels for each gametic (g)DMR in F1 mat-CD and F1 mat-HFD oocytes (merged from 41 and 37 oocyte scBS-seq datasets, respectively). b SeqMonk screenshot showing mean DNA methylation in F1 mat-CD and F1 mat-HFD oocytes over nonoverlapping 100 CpG windows (colour-coded blocks) across a ~450 kb interval encompassing the Dlk1-Dio3 imprinted cluster with a zoomed-in region (below) showing the CpG methylation calls (methylated red; un-methylated blue) of the Dlk1-Gtl2 region with quantification over the gDMR and sDMRs. Error bars represent the standard deviation from the mean of 5 pseudo-bulk groupings of 7-8 oocytes each. c Principal component analysis of scRNA-seq datasets of individual oocytes from F1 mat-CD and F1 mat-HFD . d Heatmap revealing 5 unsupervised clusters of the 166 most variable genes between F1 mat-CD and F1 mat-HFD oocytes. Top bars identify the F1 donor and diet groups. Clusters 1 to 5 comprised 25, 62, 44, 25 and 9 genes respectively. e Major terms highlighted in the gene ontology analysis of up-regulated genes from clusters 1, 2 and 4 (x-axis, -log10 of FDR adjusted p values). Gene ontology analysis was performed with GOrilla and summarised with Revigo. f Comparison of Dlk1-Dio3 microRNA (miRs) expression in F1 mat-CD (black) and F1 mat-HFD (blue) oocytes, alongside three stably expressed miRs ( 27b-3p, 103-3p, 423-3p ), analysed by small RNA sequencing. Each of the Dlk1-Dio3 miRs was found to be significantly more represented in F1 mat-HFD oocytes. (Bars represent mean counts per million ±SD; small RNA-seq libraries generated from oocytes from four female mice per group; unpaired two-sided t -tests with Holm-Šídák’s correction for multiple comparisons: ** p adj = 0.0013, *** p adj = 0.0005, **** p adj < 0.0001, ns=not significant). Source data are provided as a Source Data file. Full size image Genome-wide transcription was also examined in these F1 mat-HFD oocytes. Although PCA indicated no clear separation of oocytes according to F1 mat-CD and F1 mat-HFD groupings (Fig. 6c ), increased heterogeneity was evident in the HFD group and a subset of 166 genes showed highly variable expression (>0.528 fold from the mean standard deviation) (Fig. S9a and Supplementary Data 1 ). These genes also showed the largest differences in expression between groups (Fig. S9b ). Unsupervised hierarchical clustering segregated the variable genes into five clusters (Fig. 6d ), the largest of which (cluster 2) were more likely to be upregulated in HFD oocytes, and were associated with the regulation of translation and modulation of biosynthetic and metabolic processes (Fig. 6e ). In contrast downregulated genes did not group together in terms of function (Supplementary Data 1 ). These results show that while only limited changes in DNA methylation were seen in oocytes in response to HFD (at a genome-wide level, at the Dlk1-Dio3 cluster (Fig. 6b ), at the imprinted Ube3a locus, or a neighbouring non-imprinted locus, Atp10a (Fig. S10 )), altered transcriptional quality of oocytes from in utero HFD-exposed F1 females was readily detected. In addition, small RNA-sequencing revealed a marked increase in the expression of multiple miR species from within the Dlk1-Dio3 cluster in F1 oocytes that had been exposed to HFD, as compared to CD (Fig. 6f ). The expression of control miR species ( mir 27b-3p , mir 103-3p , mir 423-3p ) that reside outside the Dlk1-Dio3 locus, was in contrast, unchanged between F1 mat-HFD and F1 mat-CD oocyte samples. Importantly, up-regulation of Dlk1-Dio3 miRs was sustained for long periods after gestational exposure and affected clusters spanning the entire Gtl2-Rtl1as-Rian-Mirg domain (Fig. 7a ). These data show that miR expression in the developing oocytes is irrevocably altered in response to in utero exposure to HFD and implicate this in the subsequent misregulation of Dlk1 in F2 progeny. Fig. 7: Generational modulation of Dlk1-Dio3 imprinting in response to HFD exposure. a Schematic of Dlk1-Dio3 cluster miRs that were over-expressed in F1 mat-HFD oocytes, as compared to F1 mat-CD . Over-represented miRs are displayed as blue, while non-expressed miRs are displayed as grey. b Schematic summarizing the modifications to Dlk1 imprinting across generations. Imprinting is disturbed inter-generationally but restored trans-generationally. Blue (increased) and red (decreased) arrows depict expression or methylation levels relative to controls. Full size image Our study shows that dietary challenge in pregnancy, and specifically maternal exposure to HFD, induces a loss of Dlk1 imprinting that impacts two successive generations of offspring. In F1 animals, HFD-exposure provoked a sustained loss of Dlk1 imprinting in several somatic tissues, a feature that was associated with a corresponding increase in DNA methylation at the Dlk1 sDMR . In F2 animals born exclusively to F1-exposed females, Dlk1 expression was also deregulated and variable Dlk1 expression was seen among offspring, including ectopic expression in the heart. The vulnerability of F2 offspring born to F1-exposed females inferred that oocytes might be targets of exposure-induced epigenetic change. As female gametogenesis initiates in growing oocytes in the ovary postnatally [50] , [51] , [52] , any direct effect of exposure on de novo DNA methylation appeared very unlikely. Nonetheless exposure to HFD occurs contemporaneously with a widespread DNA methylation erasure in primordial germ cells of the embryo [53] , so we asked whether DNA de-methylation was impaired in F1-exposed oocytes. We saw no evidence of either residual methylation of paternal gDMRs or altered DNA methylation across the Dlk1-Dio3 domain in these oocytes. Instead, HFD-exposed F1 oocytes showed altered gene expression, detected using genome-wide scRNA-seq, including pronounced changes in expression of many Dlk1/Gtl2 -associated genes and miRs. This unexpected result suggested that two different epigenetic mechanisms are contributing to Dlk1 LOI within the developing F1 embryo and these result in distinct temporal-spatial read-outs and impacts (Fig. 7b ). Exposure to HFD in utero elicits an inappropriate expression of maternally-derived Dlk1 in several F1 somatic tissues including BAT, brain and liver, associated with increased DNA methylation at the Dlk1 sDMR . HFD-exposure also induced a de-regulated expression of miRs in developing oocytes within female F1 offspring. This is of particular interest as correct expression of Gtl2 -associated lncRNAs, miRs and snoRNAs is known to be important for restricting the expression of both maternal Gtl2 and paternal Dlk1 expression in several other contexts [54] , [55] , [56] , [57] . Mis-expression of these RNA species in individual oocytes may therefore underlie the heterogenous misregulation of Dlk1 expression that we observed in individual F2 offspring, as well as Dlk1 LOI and de novo ectopic expression of Dlk1 in cardiac tissues. The demonstration of altered miR expression in F1 oocytes is surprising given that these were sampled from F1 adults after ovulation and several weeks after HFD exposure. The results implicate an alternative (non-canonical imprinting) route of intergenerational epigenetic transmission where chromatin and miR expression, rather than DNA methylation per se, predispose Dlk1 and Gtl2 to deregulation. As histone H3K27me3 is pervasive in the oocyte genome and occupies DNA hypo-methylated domains [58] , [59] and has been shown to be responsible for a parallel imprinting mechanism [60] , [61] , it is tempting to speculate that this modification might play a role. In F1-exposed animals, we demonstrate dramatic increases in Gtl2 , Rtl1as , Rian and Mirg expression (as well as a plethora of miRs), species that are normally only expressed at low levels and exclusively from the maternal allele [24] , [27] , [62] . High levels of transcription across the Dlk1-Dio3 domain persisted in F1 animals for many months, even after being returned to a normal diet. Collectively these results offer an unanticipated explanation for the deregulation of Dlk1 seen in the next generation. As expression of miRs across the Dlk1-Dio3 domain can be self-sustaining [54] , [55] , [56] , [57] and disruption of maternally expressed miRs can alter paternal Dlk1 expression [57] , constitutive activity across this domain in oocytes would likely result in an imbalance of Dlk1 expression consistent with what is observed in F2 animals born to HFD-exposed F1 females. This study examines epigenetic mechanisms that regulate Dlk1 expression and the intergenerational mechanisms through which gestational exposure to HFD impacts imprinting at the Dlk1-Dio3 locus. While this focus on imprinting at a single locus can offer access to epigenetic regulatory mechanisms, it is worth noting that imprinting constitutes only a minor fraction of the genome. While the dietary model used here provides fresh information about how imprinting is disrupted and then conveyed to F2 offspring, further studies are needed to examine impacts at non-imprinted sites. Numerous prior studies have shown that gestational exposure to diets low in protein or high in fat impacts gene expression and metabolic circuitry in offspring [9] , [17] , [21] , [30] , [63] . While it is still unclear how maternal dietary challenges provoke long-lasting changes in offspring; methyl-donor supply, mitochondrial reprogramming, placental stress, and other mechanisms have been inferred [16] , [38] , [64] , [65] , [66] , [67] . Despite this paucity in understanding, early-life adversities such as this enhance disease risk in offspring [9] , [41] , [68] . Genome-wide studies suggest that non-imprinted genes and imprinted genes are equivalently sensitive to dietary challenge [69] , however, relatively minor changes in the expression of imprinted genes are known to provoke major changes in organismal physiology pre- and postbirth [17] , [70] . Previously we showed that exposure to low protein diet in utero results in an elevated expression of Cdkn1c in offspring, through loss of imprinting that begins mid-gestation and is retained into adulthood [30] . In this scenario, LOI was associated with reduced DNA methylation at the Cdkn1c sDMR and was partially rescued by folate supplementation. Although LPD-induced Cdkn1c LOI resulted in altered offspring behavior [40] , [71] , no obvious phenotypic changes or LOI was evident in F2 mice, in marked contrast to HFD-induced LOI observed here for Dlk1 . Several reports link maternal overnutrition to phenotypic changes in mice that span three or more generations, which are mediated through the germline, and would therefore be viewed as transgenerational [63] , [72] , [73] . These published studies have implicated sperm RNAs, miRs and tRNA-derived small RNAs in the transmission of epigenetic memory. Here we show that exposure to HFD in utero results in intergenerational epigenetic changes that are mediated through the female germline and provoke heterogenous misexpression of Dlk1 in F2 mice. As our work suggests that Dlk1 imprinting is re-instated in the subsequent F3 generation, future studies will be required to determine any transgenerational impact. Irrespective of this outcome, our study raises the intriguing possibility that genomic imprinting mechanisms that harness multiple layers of epigenetic control can enable the phenotypes of successive generations of offspring to be modified in response to environmental challenges that are precociously sampled ahead of birth. Generation of targeted ESCs and mice The Dlk1-FLucLacZ (B6NTac) line was created by Taconic Biosciences and ESCs and animal founders were delivered to Imperial College. A firefly luciferase and LacZ were knocked in to the 3’UTR of the Dlk1 gene, with T2A sites. This approach produces a single RNA, under the control of the Dlk1 promoter, in a non-disruptive manner. Upon translation the T2A sites self-cleave, liberating independent proteins of FLuc, β-galactosidase and Dlk1. Mice were back-crossed onto a B6(Cg)- Tyr c-2J /J (Jackson Labs, C57Bl/6 J albino) background for >6 generations. Maintenance of mice Mice were handled and all in vivo studies were performed in accordance with the United Kingdom Animals (Scientific Procedures) Act (1986). Mouse work was approved by the Imperial College AWERB committee and performed under a UK Home Office project license. Mice were housed on a 12-h light-dark cycle with a temperature range of 21 + /− 2 °C and a humidity range of 55 + /− 10% in pathogen-free conditions. The Dlk1-FLucLacZ line was maintained on a B6(Cg)- Tyr c-2J /J (Jackson Labs, C57Bl/6 J albino) background. For mating, males were set up with not more than three females and morning plug checking was performed. Upon plug discovery, females were considered E0.5. Genotyping of animals Genomic DNA was isolated from 4-week old ear biopsies or embryonic tails by digestion in lysis buffer (0.05 M Tris HCl pH 8, 0.025 M EDTA, 0.031% SDS, 0.02 M NaCl, 80 μg/ml Proteinase K (Sigma-Aldrich)) at 50 °C with rocking. DNA was diluted 1:2 in 10 mM Tris HCl pH8 and 1 µl of diluted DNA was used in PCR analysis (primer sequences provided below). Diet studies Dlk1-FLucLacZ females were set up with B6(Cg)- Tyr c-2J /J males and upon vaginal plug discovery, matings were separated. Females were fed either a low protein chow (5769, TestDiet), a control chow (5755, TestDiet) or a high-fat chow (45% energy from fat, 58V8, TestDiet). All animals were returned to the control diet at E18.5. Pregnant dams and embryos were imaged at E17.5 and offspring were imaged at P56. For multi-generational studies, Dlk1-FLucLacZ (males and females) mice that had been exposed to in utero HFD for the duration of pregnancy were aged to 10 weeks, with access to control diet ad libitum and set up with a B6(Cg)- Tyr c-2J /J partner. Offspring were aged to P56 prior to analysis. Bioluminescent imaging D-Luciferin (Perkin Elmer) was dissolved in H 2 0 at 30 mg/ml. Mice were weighed and injected IP with 0.15 mg/g body weight, before being anaesthetized with isofluorane. Mice were imaged 10 min postinjection, in an IVIS Spectrum (Perkin Elmer) under anaesthesia. Images of adult mice and pregnant dams were taken at field of view (FOV) C, with binning 4 and 180 s exposure. For imaging of embryos, pregnant females were injected with D-Luciferin at least 12 min prior to imaging. Embryos were dissected into 24 well dishes containing PBS and placed in the IVIS Spectrum. Images of embryos were taken at FOV A, with binning 4, focus 1 cm and 180 s exposure. No additional D-Luciferin was added, and imaging continued for up to 35 min postinjection. For ex vivo imaging of tissue, mice were culled at least 10 min after D-Luciferin injection, organs were removed and placed in clean dishes containing PBS. No further D-Luciferin was added to samples. Analysis of images was performed on Living Image software 4.5 (Caliper Life Sciences). For quantification of bioluminescent signal, regions of interest were drawn around the specified region and signal flux within the region was calculated. LacZ staining Tissues or embryos were dissected and placed in cold LacZ fixative (2% formaldehyde, 0.2% glutaraldehyde, 0.02% Nonidet P-40, 1 mM MgCl 2 , 0.1 mg/ml Sodium Deoxycholate in PBS) for 4 hr or O/N, at 4 °C with rocking. The tissue was washed in PBS, embedded in OCT (Fisher Scientific) and stored at −80 °C. Embedded tissues were sectioned (15 µm) with a CM1950 cryostat (Leica). Embryos and sectioned tissues were subsequently washed in PBS before being placed in LacZ stain (0.4 mg/ml X-Gal, 4 mM Potassium Ferrocyanide, 4 mM Potassium Ferricyanide, 1 mM MgCl 2 , 0.02% Nonidet P-40 in PBS) for 4–6 (embryos) or 24–48 (sectioned tissue) hr at 4 °C (embryos) or RT (sectioned tissue) with gentle rocking. Upon completion, embryos were washed twice in PBS before transfer to 70% ethanol and storage at 4 °C. Sectioned tissues were washed twice in PBS and mounted with coverslips and Fluoroshield containing DAPI (Insight Biotechnology). Slides were imaged with NanoZoomer-XR (Hamamatsu). Optical projection tomography LacZ stained E11.5 embryos (as above) were mounted in 2% low melting point agarose cylinders, dehydrated through graded methanol solutions and maintained in 100% methanol. For optical clearing, samples were immersed overnight in BABB (1:2 Benzyl benzoate: Benzyl alcohol, Sigma Aldrich). Optical projection tomography (OPT) was performed on an in-house low-magnification imaging system [30] , [74] . Briefly, cleared samples were suspended from a rotation stage (T-NM17A200, Zaber Technologies Inc) in a BABB-filled cuvette. Images were acquired with a CCD camera with 2 × 2 pixel binning (Clara, Andor Technology Ltd) using a telecentric zoom lens (modules NT56-625, NT59-671 and NT59-672, Edmund Optics Ltd). For LacZ stain imaging, transmitted light images were acquired through a 716 ± 20 nm band-pass filter (FF01-716/40-25, Laser 2000 UK Ltd) every 1° over a full 360° rotation. Average illumination and background images were also acquired, and these images were combined to form an integrated absorption coefficient image at each projection angle. 3D reconstructions of the absorption coefficient per voxel were produced using a filtered back-projection algorithm [75] . The whole sample volume was reconstructed from fluorescence OPT imaging with 473 nm excitation (Cobolt BluesTM, Cobolt AB) and acquisition at 520 ± 17 nm (FF01520/35-25, Laser 2000 UK Ltd). 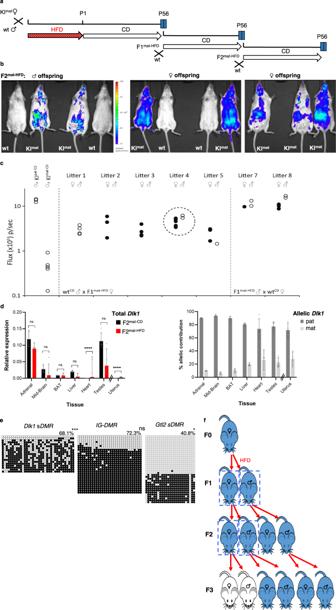Fig. 5: Exposure-induced changes toDlk1imprinting are transmitted to F2 offspring. aSchematic for generational studies following HFD exposure. Gestationally exposed animals (Dlk1-FLucLacZF1mat-HFD) were bred with wt (CD-fed) mates, maintained on CD, and F2 and F3 offspring examined.bBL signal (blue) in F2 offspring (F2mat-HFD) derived from F1 HFD-exposed females. Signal was variable and ectopic.cAbdominal BL signal in P56 F2mat-HFDmales (open-circles) and females (filled-circles), from six F1mat-HFDfemales and wtCDmales (litters 1–5, no litter from female 6) or two F1mat-HFDmales and wtCDfemales (litters 7–8). KImat-CDand KIpat-CDsignal shown for comparison. Litter 4 is represented in (b). Source data are provided as a Source Data file.dDlk1expression (QRT-PCR, left) in tissues from P56 males (uterus from females) whose mothers were exposed in utero to CD (F2mat-CD, black) or HFD (F2mat-HFD, red). Expression normalised toβ-Actin,18SandHprt(bars show geometric mean with geometric SD;N= 4 + 4 individual mice; Two-way ANOVA on delta-Ct values (Tissuep< 0.0001, Dietp= 0.002, Interactionp< 0.0001); Holm-Šídák’s multiple comparisons follow-up test for diet in each tissue: ****padj < 0.0001, ns=not significant). AllelicDlk1analysis in F2mat-HFDmice (right) showed reduced paternal (dark grey) versus maternal (light grey) expression bias, compared to control conditions (bars indicate mean allelic contribution ±SD;N= 4 + 4 individual mice). Source data are provided as a Source Data file.eBisulphite analysis in male P56 F2mat-HFDliver showedDlk1 sDMRhyper-methylation, increasedIG-DMRmethylation (padj = 0.078) and slightly reducedGtl2 sDMRmethylation, compared to F1mat-CD(Fig.4a). Closed circles: methylated CpG, open circles: un-methylated CpG. Rows show individual clones from a representative individual, percentages indicate total methylation from two animals. (Kolmogorov-Smirnov test comparing clonal methylation levels, using Holm-Šídák’s correction for multiple comparisons: *padj = 0.025, ***padj = 0.0001, ns=not significant). Source data are provided as a Source Data file.fSummary of alteredDlk1expression following gestational HFD.Dlk1is silent (white) when transmitted maternally and expressed (blue) when transmitted paternally. Gestational HFD exposure provokes LOI in F1 offspring (blue, box). F1 females transmit alteredDlk1expression to F2 offspring (blue, box), whereas F1 males and F2 females transmitDlk1appropriately. Immunostaining The tissue was dissected and fixed in ice-cold 4% PFA in PBS O/N with gentle rocking. The tissue was washed in PBS the following morning, embedded in OCT (Fisher Scientific) and stored at −80 °C. Embedded tissues were sectioned (12 µm) with a CM1950 cryostat (Leica). Sections were blocked with 10% normal goat serum (Thermo Scientific) in PBS, 0.1% Tween20 at RT for 1 h. Following blocking, samples were incubated with primary antibodies (antibody details provided below) in blocking buffer for 1 hr at RT. Samples were washed 3X in PBS, 0.1% Tween 20 for 5 mins at RT. Samples for immunofluorescence were incubated with fluorescently tagged-secondary antibodies in blocking buffer for 1 hr at RT. Samples were washed 3X in PBS, 0.1% Tween 20 for 5 mins at RT and mounted with coverslips and Fluoroshield containing DAPI (Insight Biotechnology). Images were taken with identical gain and exposure times in all instances, using a LSM880 confocal microscope (Leica). Immunofluorescence images were analysed with Zen Blue 3.4 (Zeiss). Samples for immunohistochemistry were incubated with an HRP-conjugated secondary antibody in blocking buffer for 1 h at RT. Samples were washed 3X in PBS, 0.1% Tween 20 for 5 min at RT. Samples were incubated with DAB substrate (ab64238, Abcam) for 10 min and washed 2X in PBS, 0.1% Tween 20 for 5 min at RT. Samples were counter-stained with Haematoxylin solution (Merck) for 30 s, with immediate washing 3X in PBS, 0.1% Tween 20 for 5 min at RT. Finally, samples were mounted with coverslips in mounting medium (Insight Biotechnology). Slides were imaged with NanoZoomer-XR (Hamamatsu). Immunohistochemistry images were analysed with NDP.view2 (Hamamatsu). RNA extraction and QRT-PCR analysis RNA was extracted with TRIzol (Thermo Scientific) according to manufacturer’s protocol and all RNA precipitation steps were performed with 100% ethanol. Reverse transcription was performed using Superscript III Reverse transcriptase (Invitrogen) as per the manufacturer’s protocol, with minor modifications. RT-PCR was performed on a CFX96 Real-Time System (Bio-Rad) with QuantiTect SYBR Green Master Mix (Qiagen) as per the manufacturer’s protocol, with each well pipetted in technical triplicate and each plate run in technical duplicate. Average Ct values for each biological replicate (each N ) were generated from the technical replicates. 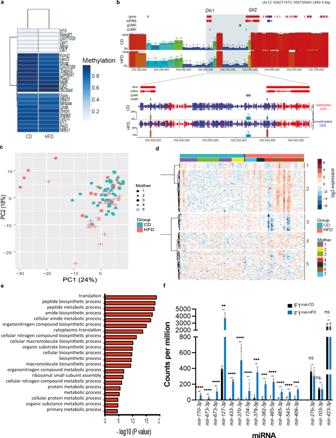Fig. 6: Germline DMRs in single MII oocytes from F1 females are unaffected by dietary exposure but show an altered transcriptional programme. aHeatmap representing mean DNA methylation levels for each gametic (g)DMR in F1mat-CDand F1mat-HFDoocytes (merged from 41 and 37 oocyte scBS-seq datasets, respectively).bSeqMonk screenshot showing mean DNA methylation in F1mat-CDand F1mat-HFDoocytes over nonoverlapping 100 CpG windows (colour-coded blocks) across a ~450 kb interval encompassing theDlk1-Dio3imprinted cluster with a zoomed-in region (below) showing the CpG methylation calls (methylated red; un-methylated blue) of theDlk1-Gtl2region with quantification over the gDMR and sDMRs. Error bars represent the standard deviation from the mean of 5 pseudo-bulk groupings of 7-8 oocytes each.cPrincipal component analysis of scRNA-seq datasets of individual oocytes from F1mat-CDand F1mat-HFD.dHeatmap revealing 5 unsupervised clusters of the 166 most variable genes between F1mat-CDand F1mat-HFDoocytes. Top bars identify the F1 donor and diet groups. Clusters 1 to 5 comprised 25, 62, 44, 25 and 9 genes respectively.eMajor terms highlighted in the gene ontology analysis of up-regulated genes from clusters 1, 2 and 4 (x-axis, -log10 of FDR adjustedpvalues). Gene ontology analysis was performed with GOrilla and summarised with Revigo.fComparison ofDlk1-Dio3microRNA (miRs) expression in F1mat-CD(black) and F1mat-HFD(blue) oocytes, alongside three stably expressed miRs (27b-3p, 103-3p, 423-3p), analysed by small RNA sequencing. Each of theDlk1-Dio3miRs was found to be significantly more represented in F1mat-HFDoocytes. (Bars represent mean counts per million ±SD; small RNA-seq libraries generated from oocytes from four female mice per group; unpaired two-sidedt-tests with Holm-Šídák’s correction for multiple comparisons: **padj = 0.0013, ***padj = 0.0005, ****padj < 0.0001, ns=not significant). Source data are provided as a Source Data file. 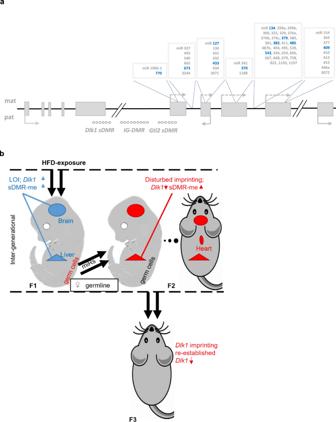Fig. 7: Generational modulation ofDlk1-Dio3imprinting in response to HFD exposure. aSchematic ofDlk1-Dio3cluster miRs that were over-expressed in F1mat-HFDoocytes, as compared to F1mat-CD. Over-represented miRs are displayed as blue, while non-expressed miRs are displayed as grey.bSchematic summarizing the modifications toDlk1imprinting across generations. Imprinting is disturbed inter-generationally but restored trans-generationally. Blue (increased) and red (decreased) arrows depict expression or methylation levels relative to controls. For relative expression, ΔCt values were calculated relative to β-Actin for comparisons within a single tissue, or using the mean of three housekeeping genes ( β-Actin, 18S, Hprt ) for multi-tissue comparisons. ΔCt values (logarithmic data, normally distributed) were used for statistical analyses, with details provided in the figure legends. The geometric means of antilog values were plotted, with error bars indicating the geometric SD. For allelic contributions, ΔCt values were calculated as ΔCt = Ct(KI mat ) – Ct(KI pat ), and converted to percentage contributions: KI pat % = 100/(2 ΔCt – 1); KI mat % = 100/(2 −ΔCt – 1). Primer sequences are provided below. Preparation of MII-oocytes Superovulation of 6-week old females was performed by evening IP injection of pregnant mare serum (PMS) followed by injection of human chorionic gonadotropin (HCG) 48 h later. The following morning, mice were sacrificed via cervical dislocation and cumulus oophorus complexes (COCs) were collected from the oviduct via mechanical dissection. After digestion with hyaluronidase (Sigma Aldrich), MII oocytes were washed in sterile PBS and collected in RLT buffer (Qiagen). Oocytes for the single-cell experiments were stored in 96-well plates at −80 °C until further processed, while oocytes for small RNA experiments were processed immediately. Single-cell bisulphite and RNA-sequencing of MII-oocytes Cell lysis was performed and Poly-A RNA was captured using oligo-dT conjugated to magnetic beads. Single-cell (sc)RNA-seq libraries were prepared according to the G&T-seq and Smartseq2 protocol [76] . The lysate containing gDNA was purified on AMPureXP beads before bisulphite-sequencing (BS-seq) libraries were prepared according to the scBS-seq protocol that has previously been described in detail [77] . Libraries were sequenced on a NextSeq500 (Illumina) with HighOutput 75 bp Paired-End (scBS-seq) or Single End (scRNA-seq) sequencing. For scBS-seq analysis, read alignment to the GRCm38 reference genome, deduplication and methylation calling was performed using Bismark v0.22.1 [78] . Oocytes with a global methylation greater than 50%, or X chromosome CGI methylation greater than 16%, were discarded from analysis. Methylation calls from all oocytes of the same group were pooled to obtain DNA methylation levels at 19 maternal gDMRs, three paternal gDMRs and two secondary DMRs. These DNA methylation levels represent the average across all CpG sites within the DMR. DMR identification from single-cell BS-sequencing was performed by pseudobulking the single oocyte datasets in groups of nine cells and quantifying DNA methylation over 100-CpG tiles to overcome the sparsity in single-oocyte data. Differential methylation was tested using a weighted logistic regression. This procedure was repeated 100 times shuffling the members of the pseudobulk groupings to avoid quantification biases. A DMR was called if the observed methylation difference was at least 10% and had an FDR < 0.05 in at least 70 of the 100 shuffling events [79] . For scRNA-seq analysis, reads were mapped with hisat2 v2.1.0 [80] against the GRCm38 reference genome and gene expression was quantified over the mouse oocyte transcriptome as log2-transformed reads per million using SeqMonk v1.46.0 ( https://www.bioinformatics.babraham.ac.uk/projects/seqmonk/ ). Principal component analysis was performed using R (R Core Team, 2016). The top variable genes were identified using the function variation plot in SeqMonk with Standard Error of the Mean parameters. Hierarchical clustering of the expression levels of the most variable genes was performed using R (R Core Team, 2016). GO analysis was done using the Gene Ontology enRIchment anaLysis and visuaLizAtion tool (GOrilla) ( http://cbl-gorilla.cs.technion.ac.il/ ) [81] , followed by reduction of terms with Revigo [ http://revigo.irb.hr ] [82] . miR analysis of MII-oocytes Total RNA was extracted from bulk oocytes with TRIzol (Thermo Scientific) according to the manufacturer’s protocol. Small RNA library preparation was performed with NEBNext Small RNA Library Prep (NEB), and microRNAs were isolated by size selection on 6% TBE PAGE gels (Novex) with clean up performed using Monarch PCR and DNA clean up kit (NEB), according to the manufacturer’s protocol. Sample validation was performed on a Bioanalyzer 2100 using High Sensitivity DNA analysis kit (both Agilent) and libraries were sequenced on a MiSeq (Illumina) and analysed using sRNAtoolbox ( https://arn.ugr.es/srnatoolbox/srnabench/ ) [83] . Clonal bisulphite sequencing (tissue) Bisulphite modification of DNA was carried out with the EZ Gold DNA Methylation Kit (Zymo Genetics) according to the manufacturer’s recommendations. PCR primers (sequences provided below) that specifically recognize bisulphite-converted DNA were used to amplify regions spanning the three imprinted DMRs associated with the Dlk1-Dio3 imprinted region, with TaKaRa EpiTaq™ HS (Takara), using the manufacturer’s protocol. PCR products were separated on an agarose gel and bands corresponding to the predicted size were excised and cleaned up with a Gel Extraction kit (QIAquick, Qiagen). Ligation of product was performed using Clone JET PCR cloning kit (Thermo Scientific) as per the manufacturer’s protocol, before transformation into DH5α cells. Bacteria were plated onto LB/Ampicillin plates and grown up overnight at 37 °C. Colonies were picked (normally 24 per sample) and expanded in LB/Ampicillin broth overnight at 37 °C. The following morning, plasmids were purified with the Wizard® SV 96 Plasmid DNA Purification System (Promega) according to the manufacturer’s protocol and sent for Sanger Sequencing (GeneWiz). Pyrosequencing (bisulphite, tissue) DNA (0.5–1 µg) was bisulphite treated using the two-step protocol of the Imprint DNA Modification Kit (Sigma). The Dlk1 sDMR region was amplified from bisulphite converted DNA through PCR with HotStarTaq DNA Polymerase (Qiagen) (primer sequences provided below). PCR products were shaken at 1,400 rpm with Streptavidin Sepharose High Performance beads (GE healthcare) in binding buffer (10 mM Tris-HCl pH7.6, 2 M NaCl, 1 mM EDTA, 0.1% Tween-20) for 20 min. The biotinylated strand of the product was purified using the PyroMark Q96 Vacuum Workstation (Qiagen). The sequencing primer was annealed to the template in annealing buffer (20 mM Tris-acetate pH7.6, 2 M magnesium acetate) at 85 °C for 4 min. Sequencing was performed with the PyroMark Q96 MD pyrosequencer (Qiagen) using PyroMark Gold Q96 Reagents (Qiagen). Bisulphite primers Clonal Dlk1 sDMR F: CCCCATCTAACTAATAACTTACA Dlk1 sDMR R: GTGTTTAGTATTATTAGGTTGGTG IG-DMR F: GTATGTGTATAGAGATATGTTTATATGGTA IG-DMR R: GCTCCATAACAAAATAATACAACCCTTCC Gtl2 sDMR F: GAAGAATTTTTTATTTGGTGAGTGG Gtl2 sDMR R: CAACACTCAAATCACCCCCC Sequencing R: CAGGAAACAGCTATGAC Pyrosequencing Dlk1 sDMR F: GTTAGAAAGGGGGTATTTGTTTTTAGTAT Dlk1 sDMR R: 5’[Btn]CTTTCATAAACACCTTCAAAATATATTACT Sequencing F: ATTTGTTTTTAGTATATTTAGGTGA QRT-PCR Primers Dlk1 F: GAAAGGACTGCCAGCACAA Dlk1 Total R: CACAGAAGTTGCCTGAGAA Dlk1 tg R: GCCGGGCCTTTCTTTATGTT Dlk1 wt R: CCCCGGTAATAGAGAAGGGC B-Actin F: CCTGTATGCCTCTGGTCGTA B-Actin R: CCATCTCCTGCTCGAAGTCT Gtl2 F: CGAGGACTTCACGCACAAC Gtl2 R: TTACAGTTGGAGGGTCCTGG Rtl1 F: TACTGCTCTTGGTGAGAGTGGACCC Rtl1 R: GGAGCCACTTCATGCCTAAGACGA Rtl1as F: TCTCCACTCGAGGGTACTCCACCT Rtl1as R: GTGGAGAACTTCGCTGTCATCGC Rian F: ATGTCTGCTGCCCTGTCGTCT Rian R: GCGGTCACTGCCAAGGTCTCT Mirg F: GTTGTCTGTGATGAGTTCGC Mirg R: GTTCTTGAACATCCGCTCC 18S F: CCTGGATACCGCAGCTAGGA 18S R: GCGGCGCAATACGAATGCCCC Hprt F: AGTGTTGGATACAGGCCAGAC Hprt R: CGTGATTCAAATCCCTGAAGT Genotyping primers Dlk1 Geno F: AGTTTGCAAGCTGCACTTGG Dlk1 Geno R: CTTTGGAGCTAGATCTTTCAGTGG Antibodies Anti-Dlk1 [3A10]: ab119930 (Abcam) Mouse monoclonal. 1:100 dilution. Antifirefly Luciferase [EPR17790]: ab185924 (Abcam) Rabbit monoclonal. 1:100 dilution. Goat antirabbit 568: A-11011 (Thermo Scientific). 1:1000 dilution. Goat antimouse 488: A-10680 (Thermo Scientific). 1:1000 dilution. Goat antimouse HRP-conjugated. #31430 (Thermo Scientific). 1:1000 dilution. Calculations, graphs and statistical analysis Microsoft Excel and GraphPad Prism (v9.2.0) were used for calculations, statistical analysis and the preparation of graphs. In general, figures show the mean and standard deviation or geometric mean and geometric standard deviation, with details provided in the figure legends. Data were tested for normality prior to statistical tests where relevant (D’Agostino-Pearson omnibus K2), and statistical tests were performed on log-transformed data (delta-Ct values for QRT-PCR data) where appropriate, as indicated in the figure legends. Multi-group comparisons were generally tested by One-way or Two-Way ANOVA, followed by either Dunnett’s (comparisons to control only) or Holm-Šídák’s (comparisons between each group) two-sided multiple comparisons follow-up tests. For experiments where pair-wise comparisons were determined a priori, unpaired two-sided t-tests with Holm-Šídák’s correction for multiple comparisons were performed directly. DNA bisulphite data were compared using the Kolmogorov-Smirnov test (comparing clonal methylation levels), using Holm-Šídák’s correction for multiple comparisons. Specific details of statistical tests and results are provided in the figure legends. Raw data and output from statistical analyses are provided in the Source Data file. Reporting summary Further information on research design is available in the Nature Research Reporting Summary linked to this article.